Divergent paths for the selection of immunodominant epitopes from distinct antigenic sources Immunodominant epitopes are few selected epitopes from complex antigens that initiate T-cell responses. Here to provide further insights into this process, we use a reductionist cell-free antigen-processing system composed of defined components. We use the system to characterize steps in antigen processing of pathogen-derived proteins or autoantigens and we find distinct paths for peptide processing and selection. Autoantigen-derived immunodominant epitopes are resistant to digestion by cathepsins, whereas pathogen-derived epitopes are sensitive. Sensitivity to cathepsins enforces capture of pathogen-derived epitopes by major histocompatibility complex class II (MHC class II) before processing, and resistance to HLA-DM-mediated-dissociation preserves the longevity of those epitopes. We show that immunodominance is established by higher relative abundance of the selected epitopes, which survive cathepsin digestion either by binding to MHC class II and resisting DM-mediated-dissociation, or being chemically resistant to cathepsins degradation. Non-dominant epitopes are sensitive to both DM and cathepsins and are destroyed. Immunodominance is a well-established phenomenon whereby a few specific peptides are selected as representative epitopes of a given protein antigen to the immune system. A restricted response to an antigen might be necessary for keeping the sheer number of memory T cells within a narrow range that can be accommodated by lymph nodes, as a portion of memory T cells are maintained throughout life [1] . Many studies have aimed to understand mechanisms of epitope selection and immunodominance; a range of hypotheses related to the structural features of antigens [2] , [3] , [4] , sensitivity to proteases [5] , [6] , epitope affinity for major histocompatibility complex (MHC) class II [7] , T-cell precursor frequency [8] and T-cell receptor affinity for peptide/MHCII [9] have been considered. These studies suggest that the mechanisms evolved for the selection of the dominant epitopes are rather complex. Antigen presentation to CD4 + T cells by antigen-presenting cells (APCs) begins by the uptake of exogenous antigens and their processing that involves transfer through a series of endosomal compartments containing suitable denaturing environment, accessory chaperones and cathepsins [10] . Newly synthesized MHCII molecule associates with the class II invariant chain (Ii), which targets it to specialized endosomal compartments (MIIC) where the Ii is proteolysed until only a fragment known as the class II-associated invariant chain peptide (CLIP) remains bound in the MHCII peptide-binding groove. Efficient displacement of CLIP from the MHC groove requires the accessory molecule HLA-DM in human or H2-M in mice (DM) [11] . DM functions by inducing conformational changes in MHCII/peptide complexes resulting in the release of the bound peptide inducing a peptide-receptive MHCII [12] . A peptide-receptive MHCII can quickly sample a large pool of peptides derived from exogenously acquired proteins and DM helps in shaping epitope selection. The molecular detail of the interactions between DM and MHCII hints at a critical role for DM in selection of immunodominant epitopes [13] . However, this role has not been fully evaluated. Importantly, there is no consensus as to when immunodominant epitopes are selected. It is not clear at what stage during this process DM exerts its function. The question is whether epitopes are first cut by the antigen-processing enzymes and then captured, or epitopes bind to MHCII as full-length proteins or large fragments, and are then processed. Different cathepsins and the proper microenvironment to support their functions are provided in the MIIC [14] . Multiple studies using protease inhibitors in combination with protease-deficient Tg mice revealed that several enzymes, including cathepsins (Cat) S, L and F might contribute to antigen processing and the removal of CLIP [15] . Asparaginyl endopeptidase (AEP), present in the late endosomal compartments, is necessary for the cleavage and activation of cathepsins [16] ; although a role for generation, as well as destruction of antigenic epitopes by AEP have also been reported [17] . To directly address specific questions regarding steps in antigen processing and the selection of immunodominant epitopes, we have developed a reductionist antigen-processing system for MHCII molecules that incorporates defined components and accurately predicts immunodominant epitopes from protein antigens [18] . The system includes soluble purified HLA-DR (DR), CatB, CatH and CatS that process protein antigens into peptides, and DM. Mass spectrometry is used for sequencing the unique peaks derived from each protein. Candidate epitopes are verified for accuracy in DR transgenic mice and humans [18] . Due to the defined molecular composition, this system lends itself to elucidating steps involved in antigen processing and the roles individual components play in epitope selection. In this study, we addressed the determinants of immunodominance. We report that immunodominant epitopes from different antigenic sources are selected based on their relative abundance that rely on differential sensitivity to cathepsins, or resistance to DM-mediated dissociation. CA-074ME inhibits processing of type II collagen and H5N1-HA Cysteine proteases are a major family of intracellular proteases best studied in antigen processing by APCs. As mentioned above, CatB, H and S are the only proteases in our cell-free antigen-processing system. To test their roles in dominant epitope selections in cells, we used a cell-permeable CatB inhibitor, CA-074ME during the processing and presentation of type II collagen and H5N1-HA proteins ex vivo . While CA-074 is a potent inhibitor of CatB, addition of methyl ester group to make it cell permeable has made it a partial inhibitor of CatS as well. However, on entry into the cell, the methyl ester group is lost and the remarkable potency of CA-074 as CatB inhibitor is revealed [19] . Specific T cells were generated in DR1 (DRB1*0101) transgenic mice by immunization with type II collagen (CII) derived-epitope CII(280–294), or H5N1-HA-derived epitope, H5N1-HA(259–274), in complete Freund’s adjuvant (CFA). Cells from draining lymph nodes were cultured in the presence of either peptides, or proteins in the presence or absence of the inhibitors. As shown in Fig. 1 and Supplementary Fig. 1 , addition of CA-074ME in control groups did not affect the presentation of CII and H5N1-HA-derived epitopes as measured by interferon-γ (IFN-γ) enzyme-linked immunospot (ELISPOT) assay. In contrast, in the presence of CA-074ME, processing and presentations of both proteins were completely inhibited. These results confirm that cathepsin B is a crucial component of antigen processing for the generation of CII(280–294) or HA(259–274) dominant epitopes. 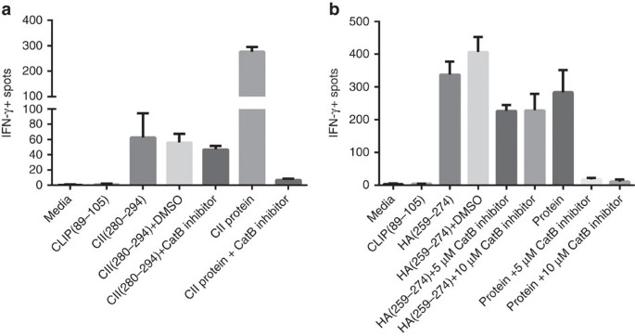Figure 1: Cathepsin B is a critical endosomal protease for generation of CII(280–294) and H5N1-HA(259–274) immunodominant epitope. ELISPOT assay measuring IFN-γ production of T cells isolated from DR1-transgenic mice immunized with CII(280–294) (a), or H5N1-HA(259–274) (b) in CFA. Cells were stimulated with peptides or proteinsin vitrofor 24 (a) or 48 h (b) in the presence or absence of cell-permeable cathepsin B inhibitor, CA-074ME. Data shown here are representative of three independent experiments. Error bars are defined as s.d. Figure 1: Cathepsin B is a critical endosomal protease for generation of CII(280–294) and H5N1-HA(259–274) immunodominant epitope. ELISPOT assay measuring IFN-γ production of T cells isolated from DR1-transgenic mice immunized with CII(280–294) ( a ), or H5N1-HA(259–274) ( b ) in CFA. Cells were stimulated with peptides or proteins in vitro for 24 ( a ) or 48 h ( b ) in the presence or absence of cell-permeable cathepsin B inhibitor, CA-074ME. Data shown here are representative of three independent experiments. Error bars are defined as s.d. Full size image DM alone is not sufficient for selection of CII(280–294) DM has been proposed as a critical component of the antigen-processing machinery contributing to the selection of the immunodominant epitopes [20] . To evaluate this notion, we used our reductionist system for the selection of the known DR1-restricted immunodominant epitope of bovine CII (bCII) [21] . Generation of this epitope involves prior digestion by gelatinase B (MMP-9). A comparison of mass spectra from five samples incorporating MMP-9 pre-cut bCII [18] with all or selected components in the system is shown in Fig. 2 . Samples a–d contained MMP-9-digested bCII peptide mixtures whereas sample e served as the background lacking bCII (unabridged spectra are shown in Supplementary Fig. 2 ). The known immunodominant bCII peptide appeared as a cluster of variants with different post-translational modifications ( Fig. 2a–d ) and was absent from all background control experiments missing the CII fragments ( Fig. 2e and Supplementary Fig. 2e–h ). Other CII-derived epitopes (shown in blue in Fig. 2a–d ) were also detected in samples including DR with either DM or cathepsins ( Fig. 2a–c ). However, those epitopes disappeared only when all the components were present ( Fig. 2d ). The two most prominent CII-derived peptides at m/z 1,413 and 1,435 Da were sodiated and non-sodiated forms of the same peptide, bCII(954–968) 2OH ( Fig. 2a–c ). To assess the immunogenicity of these epitope in mice, DR1-transgenic mice were immunized with CII protein in CFA and cells from draining lymph nodes were cultured in the presence of either peptide. As shown in Fig. 2f , cells responded to the dominant epitope as measured by T-cell proliferation and interleukin-2 (IL-2) production, but did not respond to CII(954–968) 2OH peptide, suggesting that CII(954–968) 2OH is not an immunogenic epitope. To confirm the sensitivity of CII(954–968) 2OH and of the immunodominant epitope to DM, we measured the dissociation kinetics of fluorescein-labelled CII(954–968) 2OH and CII(280–294) in complex with DR1 in the presence or the absence of DM. FL-CII(954–968) 2OH peptide showed sensitivity to DM-mediated dissociation ( Fig. 2g ). Against our expectations, the CII dominant epitope also showed sensitivity to DM-mediated dissociation ( Fig. 2h ). 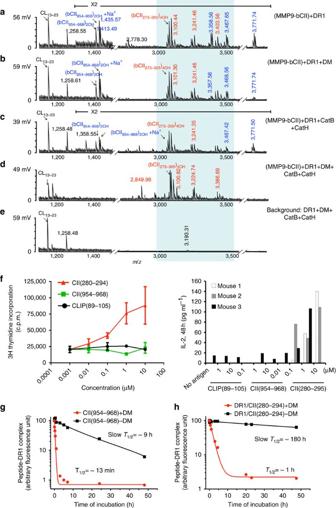Figure 2: Cathepsins and HLA-DM are necessary for the selection of the immunodominant epitope of type II collagen. (a–d) Mass spectra of peptides eluted from DR1 containing MMP-9-fragmented bCII. (e) The negative control reactions that do not contain the antigen. DR1 used in all experiments shown here (except for in sampled) was preincubated with HA(Y308A) to forms short-lived complexes with DR1(DR1/HA(Y308A) (T1/2~34 min) to induce a peptide-receptive conformation23. Them/z1,258 Da peak seen ineis background peptide peak of an insect-derived protein that binds to a portion of purified DR1 and is present in most DR1 preparations. The peaks in the shaded area represent post-translationally modified variants of a dominant peptide composed of residues 273–305 of bCII (QTGEPGIAGFKGEQGPKGEPGPAGVQGAPGPAG). Mass species in red represent CII-derived peptides containing the immunodominant core CII(282–289). Non-dominant peptides are shown in blue. Background peptide species are labelled in black. These experiments were repeated more than three times. The experiments were performed either with two cathepsins only or all three with similar results. (f) Proliferation of T cells isolated from DR1-transgenic mice immunized with bCII protein in CFA in response to stimulation with, CII(280–294), CII(954–968) or CLIP(89–105)in vitro. Cellular proliferation was measured by [3H] thymidine incorporation (left panel). The data shown here are a representative result of one mouse out of four individual mice tested. Error bars are defined as s.d. IL-2 ELISA was performed from supernatant collected fromin vitroculture of another three individual mice immunized with CII protein/CFA. Cell culture supernatants were removed after 48 h culture (right panel). (g,h) Dissociation assay of fluorescently labelled non-dominant epitope, CII(954–968) and immunodominant epitope CII(280–294) from DR1. Fluorescently labelled CII(954–968)/DR1 complexes (g) or fluorescently labelled CII(280–294)/DR1 complexes (h) were dissociated in the presence of 100 μM of unlabelled HA(306–318) at 37 °C for the indicated times in the absence (square) or presence of DM (circle). The fluorescence of the labelled complex before dissociation is arbitrarily assigned a value of 100, and fluorescence after dissociation is expressed as a fraction of fluorescence before dissociation. Representative of three dissociation experiments. Figure 2: Cathepsins and HLA-DM are necessary for the selection of the immunodominant epitope of type II collagen. ( a – d ) Mass spectra of peptides eluted from DR1 containing MMP-9-fragmented bCII. ( e ) The negative control reactions that do not contain the antigen. DR1 used in all experiments shown here (except for in sample d ) was preincubated with HA(Y308A) to forms short-lived complexes with DR1(DR1/HA(Y308A) ( T 1/2 ~34 min) to induce a peptide-receptive conformation [23] . The m/z 1,258 Da peak seen in e is background peptide peak of an insect-derived protein that binds to a portion of purified DR1 and is present in most DR1 preparations. The peaks in the shaded area represent post-translationally modified variants of a dominant peptide composed of residues 273–305 of bCII (QTGEPGIA GFKGEQGPK GEPGPAGVQGAPGPAG). Mass species in red represent CII-derived peptides containing the immunodominant core CII(282–289). Non-dominant peptides are shown in blue. Background peptide species are labelled in black. These experiments were repeated more than three times. The experiments were performed either with two cathepsins only or all three with similar results. ( f ) Proliferation of T cells isolated from DR1-transgenic mice immunized with bCII protein in CFA in response to stimulation with, CII(280–294), CII(954–968) or CLIP(89–105) in vitro . Cellular proliferation was measured by [ 3 H] thymidine incorporation (left panel). The data shown here are a representative result of one mouse out of four individual mice tested. Error bars are defined as s.d. IL-2 ELISA was performed from supernatant collected from in vitro culture of another three individual mice immunized with CII protein/CFA. Cell culture supernatants were removed after 48 h culture (right panel). ( g , h ) Dissociation assay of fluorescently labelled non-dominant epitope, CII(954–968) and immunodominant epitope CII(280–294) from DR1. Fluorescently labelled CII(954–968)/DR1 complexes ( g ) or fluorescently labelled CII(280–294)/DR1 complexes ( h ) were dissociated in the presence of 100 μM of unlabelled HA(306–318) at 37 °C for the indicated times in the absence (square) or presence of DM (circle). The fluorescence of the labelled complex before dissociation is arbitrarily assigned a value of 100, and fluorescence after dissociation is expressed as a fraction of fluorescence before dissociation. Representative of three dissociation experiments. Full size image The above findings prompted a hypothesis that DM-sensitive non-dominant epitopes are dissociated by DM and are digested away by the cathepsins, while the dominant epitopes, despite sensitivity to DM, survive the enzymatic digestion and emerge as dominant. To verify this hypothesis, we preincubated CII fragments with cathepsins for 3 h, 1 h or 15 min before adding DR1 and DM, or mixed together all the components at once. 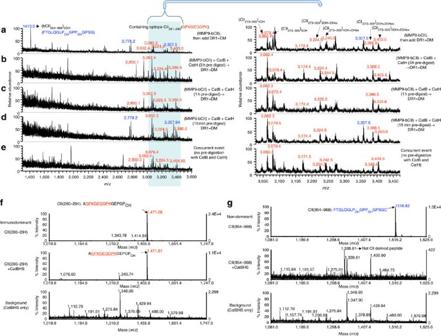Figure 3: Type II collagen-derived immunodominant peptides are resistant to cathepsin digestion. (a–e) Mass spectra of peptides eluted from DR1 are shown form/zrange of 1,400–3,600 Da. (a) MMP-9-bCII was incubated with DR1 and DM for 3 h. (b) MMP-9-bCII was first exposed to cathepsins B and H for 3 h, (c) for 1 h or (d) for 15 min, and then incubated with DR1 and DM for additional 3 h. (e) Mass spectrum of peptides eluted from DR1 when all components of the cell-free assay were mixed simultaneously and incubated together for 3 h. As inFig. 2, the peaks in the shaded area between 3,000 and 3,550 Da represent post-translational modification variants of the dominant peptide bCII(273–305). Immunodominant peptides are labelled in red and non-dominant CII peptides are shown in blue. CII protein predigestion assays were repeated three times. (f) Mass spectra of synthetic CII(280–294) immunodominant peptide and (g) Mass spectra of synthetic non-dominant CII(954–968) that were directly exposed to the cathepsins, B, H and S for 1 h at 37 °C. Top spectra in bothfandgshow synthetic peptides without treatment. Middle spectra show samples incubated with the cathepsins. Bottom spectra correspond to the background samples containing only cathepsins. The peak atm/z1,338 Da of the middle spectrum in (g) is not derived from the collagen CII(954–968); it is a background peptide from cathepsins. These experiments were repeated three times. Figure 3a–e indicates that the clusters of peptides containing the core dominant epitope ( m/z 3,000–3,500 Da range) were present regardless of the length of exposure to the cathepsins. However, when all the components were present, cathepsin-sensitive epitopes (shown in blue) were digested away ( Fig. 3e ). To further evaluate these findings, synthetic dominant CII(280–294) ( Fig. 3f ) and non-dominant CII(954–968) 2OH ( Fig. 3g ) peptides were directly exposed to the cathepsins. The dominant epitope was prominently detected at m/z 1,471 Da after exposure to cathepsins ( Fig. 3f , middle), whereas the non-dominant peptide was no longer detectable ( Fig. 3g , middle). A new peptide peak that appeared at m/z 1,338 Da was sequenced and was not a CII(954–968) 2OH derived peptide ( Fig. 3g , middle). These observations indicate that complexes of DR1/CII immunodominant epitope are sensitive to DM-mediated dissociation but resistant to degradation by cathepsins. Figure 3: Type II collagen-derived immunodominant peptides are resistant to cathepsin digestion. ( a – e ) Mass spectra of peptides eluted from DR1 are shown for m/z range of 1,400–3,600 Da. ( a ) MMP-9-bCII was incubated with DR1 and DM for 3 h. ( b ) MMP-9-bCII was first exposed to cathepsins B and H for 3 h, ( c ) for 1 h or ( d ) for 15 min, and then incubated with DR1 and DM for additional 3 h. ( e ) Mass spectrum of peptides eluted from DR1 when all components of the cell-free assay were mixed simultaneously and incubated together for 3 h. As in Fig. 2 , the peaks in the shaded area between 3,000 and 3,550 Da represent post-translational modification variants of the dominant peptide bCII(273–305). Immunodominant peptides are labelled in red and non-dominant CII peptides are shown in blue. CII protein predigestion assays were repeated three times. ( f ) Mass spectra of synthetic CII(280–294) immunodominant peptide and ( g ) Mass spectra of synthetic non-dominant CII(954–968) that were directly exposed to the cathepsins, B, H and S for 1 h at 37 °C. Top spectra in both f and g show synthetic peptides without treatment. Middle spectra show samples incubated with the cathepsins. Bottom spectra correspond to the background samples containing only cathepsins. The peak at m/z 1,338 Da of the middle spectrum in ( g ) is not derived from the collagen CII(954–968); it is a background peptide from cathepsins. These experiments were repeated three times. Full size image Dominant epitopes of HA1 are sensitive to cathepsins To test if the CII results were applicable to other antigens, we used a well-known epitope from A/Texas/1/77 influenza strain, HA(306–318) [18] , [22] . Contradictory to CII predigestion data, nearly all recombinant influenza hemagglutinin (rHA1)-derived peptides were degraded by pre-exposure to cathepsins for 3 h ( Fig. 4a ). Few rHA1-derived peptides were detectable (shown in blue) after 1 h, or 15 min exposure, but HA(306–318)-containing epitope was not found under any condition tested ( Fig. 4b,c ). Peptides containing the immunodominant epitope were identified only when all components were mixed together ( Fig. 4d , highlighted in red) or when the order of reactions were changed to the incubation of full-length rHA1 protein with DR1 and DM first, then adding the cathepsin mix ( Fig. 4e ). Other rHA1-derived peptides were also observed at m/z 1,955, 2,102, 2,265 and 2,339 Da (highlighted in blue). We surmised that the successful generation of immunodominant peptides from rHA1 protein depends on its capture by DR and editing by DM before the proteolytic fragmentation of the antigen. These data suggest a different temporal relationship between epitope capture and processing for HA versus CII proteins. 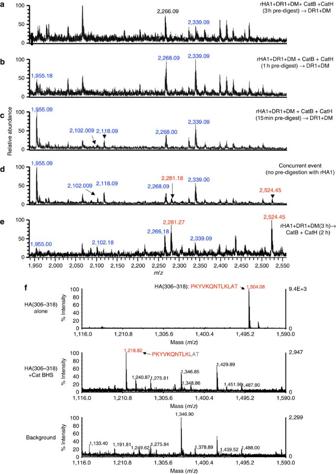Figure 4: Degradation of HA(306–318) by the cathepsins outcompetes its capture by HLA-DR1. (a–e) The mass spectra of peptides eluted from DR1. Mass species in red represent rHA1 fragments containing the DR1-restricted immunodominant HA(306–318) epitope. Peptides highlighted in blue represent other rHA1-derived peptides eluted from DR1. Recombinant HA1 was first exposed to cathepsins B and H for (a) 3 h, (b) 1 h or (c) 15 min, followed by incubation with DR1 and DM for 2 h at 37 °C. (d) Mass spectrum of peptides eluted from DR1 when all components were mixed simultaneously and incubated together for 3 h. (e) Mass spectra of peptides eluted from DR1 when rHA1 was incubated with DR1 and DM for 3 h first, and then incubated with the cathepsins for additional 2 h. (f) Sensitivity of synthetic HA(306–318) to the cathepsins tested by direct exposure to cathepsins B, H and S. Top spectrum shows HA(306–318) peptide alone. Middle spectrum is the sample reaction containing HA(306–318) incubated with the cathepsins for 1 h at 37 °C and the bottom spectrum shows the background sample containing the cathepsin mix without the synthetic peptide. Experiments were repeated three times. Figure 4: Degradation of HA(306–318) by the cathepsins outcompetes its capture by HLA-DR1. ( a – e ) The mass spectra of peptides eluted from DR1. Mass species in red represent rHA1 fragments containing the DR1-restricted immunodominant HA(306–318) epitope. Peptides highlighted in blue represent other rHA1-derived peptides eluted from DR1. Recombinant HA1 was first exposed to cathepsins B and H for ( a ) 3 h, ( b ) 1 h or ( c ) 15 min, followed by incubation with DR1 and DM for 2 h at 37 °C. ( d ) Mass spectrum of peptides eluted from DR1 when all components were mixed simultaneously and incubated together for 3 h. ( e ) Mass spectra of peptides eluted from DR1 when rHA1 was incubated with DR1 and DM for 3 h first, and then incubated with the cathepsins for additional 2 h. ( f ) Sensitivity of synthetic HA(306–318) to the cathepsins tested by direct exposure to cathepsins B, H and S. Top spectrum shows HA(306–318) peptide alone. Middle spectrum is the sample reaction containing HA(306–318) incubated with the cathepsins for 1 h at 37 °C and the bottom spectrum shows the background sample containing the cathepsin mix without the synthetic peptide. Experiments were repeated three times. Full size image To validate cathepsin sensitivity of the dominant epitope of rHA1, synthetic HA(306–318) was exposed to the cathepsin mixture. Compared with the sample containing only HA(306–318) at m/z 1,504 Da ( Fig. 4f , top), cathepsin-exposed HA(306–318) became shorter and appeared at m/z 1,218 Da. It was sequenced as PKYVKQNTLK missing LAT at its carboxyl terminus (C terminus) ( Fig. 4f , middle). To test PKYVKQNTLK for binding to DR1, peptide HA(306–318) was exposed to cathepsins before incubation with peptide-receptive DR1 (ref. 23 ) and the bound peptides were eluted and assessed by mass spectrometry. While the parallel control peptide HA(306–318) was detected, the short peptide HA(306–315) was not found likely due to the inability to bind DR1. In that sample, only the bacculovirus-derived background peptide CL(13–23) that co-purifies with DR1 was detected ( Supplementary Fig. 3a , middle). Sensitivity of the HA(306–318) peptide to degradation by the cathepsins was further tested by a cellular read out using Clone 1 T cells (CL-1) specific for HA(306–318)/HLA-DR1 (refs 24 , 25 ) HA(306–318) peptide was incubated with cathepsin mix, cathepsins were heat-inactivated and the sample was used to pulse DR1 + Epstein–Barr virus-transformed B cells as APCs. The peptide subjected to digestion did not activate CL-1 T cells, whereas the control peptide, HA(306–318) without prior cathepsin digestion did ( Supplementary Fig. 3b ). All the experiments above establish that HA(306–318) is sensitive to cathepsin digestion. We next examined immunodominant epitope from rHA1 of H5N1 strain of influenza, HA(259–274) (ref. 18 ) and obtained similar results as above. 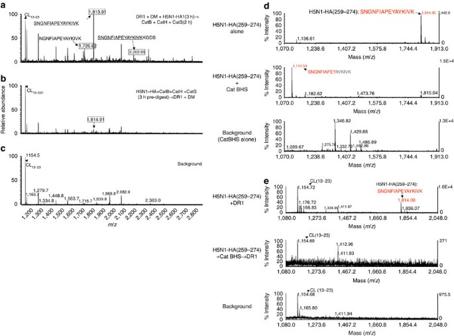Figure 5: Immunodominant epitope of H5N1-rHA1 is sensitive to the cathepsins. (a–c) The mass spectra of peptides eluted from DR1 when (a) denatured H5N1-rHA1 (A/Vietnam/1203/2004) was first incubated with DR1 and DM, and then exposed to cathepsins B, H and S or (b) when denatured H5N1-rHA1 was first exposed to the cathepsins for 3 h and then incubated with DR1 and DM. (c) The background spectrum. Boxed mass species represent H5N1-rHA1 fragments containing the DR1-restricted immunodominant HA(259–274) epitope. (d,e) mass spectra of the synthetic HA(259–274). (d) Similar to the procedure inFig. 4f, the top panel shows undigested HA(259–274) peptide. Digested peptide with the cathepsins is shown in the middle panel, and the bottom panel shows cathepsins alone as a background control. (e) Mass spectra of peptides eluted from DR1, after 3 h incubation of DR1 with HA(259–274) peptide alone (top), HA(259–274) digested with the cathepsins (middle), or the cathepsins alone (bottom). Baculovirus-derived peptide CL(13–23) was detected in every spectra from samples containing DR1. Experiments were repeated three times. Figure 5a shows that when H5N1-rHA1 protein was incubated with DR1 and DM first, followed by cathepsin digestion, unique peptide species were detected at m/z 1,726, 1,813 and 2,202 Da that shared the same core dominant epitope. When H5N1-rHA1 was first digested with cathepsins, a significantly lower peak intensity at m/z 1,814 Da emerged, and the peptides at m/z 1,726 and 2,202 Da were no longer present ( Fig. 5b ) indicating that this epitope might be susceptible to cathepsin digestion. Next, the sensitivity of H5N1-rHA1 dominant epitope, HA(259–274), to cathepsins was examined ( Fig. 5d,e ). A shorter peptide, SNGNFIAPEY, missing four amino acids from the C terminus of HA(259–274), emerged as a major peak at m/z 1,111 Da ( Fig. 5d , middle). Only a trace of the undigested peptide was detected at m/z 1,815 Da ( Fig. 5d , middle). In a parallel set of experiments, when HA(259–274) was digested with the cathepsins before incubation with DR1, no trace of the HA(259–274) was detected and only the bacculovirus-derived background peptide was found ( Fig. 5e ). The short peptide detected at m/z 1,111 Da ( Fig. 5d , middle) was not captured by DR1 ( Fig. 5e , middle). This again demonstrates that H5N1-HA-derived HA(259–274) epitope is sensitive to degradation by the cathepsins in the system, hence protein binding to DR1 should precede peptide generation to protect this epitope from fast degradation by the cathepsins. Thus far, we have shown that CII dominant epitope is sensitive to DM-mediated dissociation but resistant to cathepsin digestion. On the contrary, HA-derived dominant epitopes both showed full sensitivity to cathepsins. However, both HA-derived epitopes are insensitive to DM-mediated dissociation [26] . Hence, not all antigens are processed similarly; some bind MHC class II first, and then are processed, while some others are processed into short peptides first and then bind to MHC class II. Figure 5: Immunodominant epitope of H5N1-rHA1 is sensitive to the cathepsins. ( a – c ) The mass spectra of peptides eluted from DR1 when ( a ) denatured H5N1-rHA1 (A/Vietnam/1203/2004) was first incubated with DR1 and DM, and then exposed to cathepsins B, H and S or ( b ) when denatured H5N1-rHA1 was first exposed to the cathepsins for 3 h and then incubated with DR1 and DM. ( c ) The background spectrum. Boxed mass species represent H5N1-rHA1 fragments containing the DR1-restricted immunodominant HA(259–274) epitope. ( d , e ) mass spectra of the synthetic HA(259–274). ( d ) Similar to the procedure in Fig. 4f , the top panel shows undigested HA(259–274) peptide. Digested peptide with the cathepsins is shown in the middle panel, and the bottom panel shows cathepsins alone as a background control. ( e ) Mass spectra of peptides eluted from DR1, after 3 h incubation of DR1 with HA(259–274) peptide alone (top), HA(259–274) digested with the cathepsins (middle), or the cathepsins alone (bottom). Baculovirus-derived peptide CL(13–23) was detected in every spectra from samples containing DR1. Experiments were repeated three times. Full size image Protein binds to MHC class II molecules If the processing of antigen takes place after the binding of antigen to DR1, a complex of protein with MHC class II molecule should be detectable. To test this notion, we used a gentle SDS-polyacrylamide gel electrophoresis (PAGE) assay originally used to detect peptide binding to MHC class II in which samples were not boiled [27] , [28] . Binding of full-length rHA1 protein to DR1 was detected by its slower migrating molecular species in the presence of DR1, rHA1 and DM ( Fig. 6a , lane7, and Fig. 6b lane 4 and 6). Importantly, Fig. 6b shows that the molecular mass of the DR1/rHA1 protein complex was estimated to be ~96 kD (marked by *), that is, the sum of rHA1 (~45 kD marked by ) and DR1 alone (~51 kD; lane 2). In the presence of excess HA(306–318) in the reaction, the band intensity at ~96 kD was significantly reduced ( Fig. 6b , lane 8 and lane 17) and the new band that appeared matched the migration pattern of HA(306–318)/DR1 complex (marked by ) ( Fig. 6b , lane8, lane 9). These data indicate that the interaction with HA1 protein occurred specifically through the peptide-binding groove of DR1. Consistent with the role for DM in generating the peptide-receptive conformation of DR molecules, inclusion of DM together with DR1 and the rHA1 proteins resulted in more intensely stained bands corresponding to the protein/DR1 complexes ( Fig. 6a , lanes 6 and 7, and in Fig. 6b lanes 4, 6, 15 and 16). 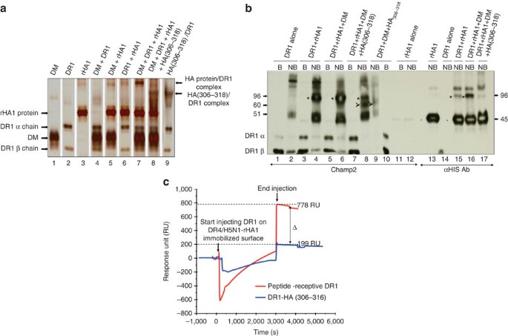Figure 6: Intact protein antigens form complexes with HLA-DR. (a,b) SDS-stable complex formation with intact proteins and DR1. Various combinations of DR1, DM, rHA1 and synthetic HA(306–318) peptide were incubated in citrate-phosphate buffer pH 5.0 for 2 h at 37 °C. Different combinations of proteins and peptides (shown in different lanes) were analysed by ‘gentle’ SDS-PAGE in which samples are not boiled before loading and (a) silver-stained or (b) western blotted. Polyclonal anti-DR1 serum (CHAMP2) or anti-His antibody was used for detecting protein/DR complexes in (b). Recombinant HA1 protein/DR1 complexes (marked by *) migrated at approximately 96 kD molecular mass. Unbound rHA1 protein migrated at ~45 kD (marked by >), HA(306–318)/DR1 migrated at around 60 kD (marked by ), and DR1 is shown at about 50 kD. B, boiled, NB, non-boiled. rHA1/DR1 complexes were estimated to migrate at 96 kD molecular mass in bothaandb. (c) Simultaneous binding of two DR alleles to H5N1-rHA1 protein as detected by BIAcore. Biotinylated DR4/HA(Y308A) complex was incubated with denatured H5N1-rHA1 protein for 20 min at 37 °C in the presence of DM, during which HA(Y308A) would dissociate and be replaced by H5N1-HA1 protein. At the end of the incubation, DR4/H5N1-rHA1 protein complex was injected over the streptavidin-coated sensor chip (SA) for 600 s and produced 3,500 RU, shown as time zero. Then, receptive DR1 (preincubated with HA(Y308A) (red) or closed HA(306–318) complex (as control) (blue) were injected over H5N1-rHA1 bound DR4 immobilized surface in the presence of DM for 3,000 s after which running buffer was injected over the chip to monitor the binding of proteins. Sensograms from both injections are superimposed in the figure for comparison. Negative sensograms observed during the injection are due to changes in buffer conditions between the running buffer and the sample buffer. Binding of the protein of interest to the immobilized protein are shown in the Response Unit (RU) indicating the RU difference between the injection start time versus injection end time. Figure 6: Intact protein antigens form complexes with HLA-DR. ( a , b ) SDS-stable complex formation with intact proteins and DR1. Various combinations of DR1, DM, rHA1 and synthetic HA(306–318) peptide were incubated in citrate-phosphate buffer pH 5.0 for 2 h at 37 °C. Different combinations of proteins and peptides (shown in different lanes) were analysed by ‘gentle’ SDS-PAGE in which samples are not boiled before loading and ( a ) silver-stained or ( b ) western blotted. Polyclonal anti-DR1 serum (CHAMP2) or anti-His antibody was used for detecting protein/DR complexes in ( b ). Recombinant HA1 protein/DR1 complexes (marked by *) migrated at approximately 96 kD molecular mass. Unbound rHA1 protein migrated at ~45 kD (marked by >), HA(306–318)/DR1 migrated at around 60 kD (marked by ), and DR1 is shown at about 50 kD. B, boiled, NB, non-boiled. rHA1/DR1 complexes were estimated to migrate at 96 kD molecular mass in both a and b . ( c ) Simultaneous binding of two DR alleles to H5N1-rHA1 protein as detected by BIAcore. Biotinylated DR4/HA(Y308A) complex was incubated with denatured H5N1-rHA1 protein for 20 min at 37 °C in the presence of DM, during which HA(Y308A) would dissociate and be replaced by H5N1-HA1 protein. At the end of the incubation, DR4/H5N1-rHA1 protein complex was injected over the streptavidin-coated sensor chip (SA) for 600 s and produced 3,500 RU, shown as time zero. Then, receptive DR1 (preincubated with HA(Y308A) (red) or closed HA(306–318) complex (as control) (blue) were injected over H5N1-rHA1 bound DR4 immobilized surface in the presence of DM for 3,000 s after which running buffer was injected over the chip to monitor the binding of proteins. Sensograms from both injections are superimposed in the figure for comparison. Negative sensograms observed during the injection are due to changes in buffer conditions between the running buffer and the sample buffer. Binding of the protein of interest to the immobilized protein are shown in the Response Unit (RU) indicating the RU difference between the injection start time versus injection end time. Full size image Simultaneous binding of two DR alleles to H5N1-rHA1 If the full-length proteins bind to MHC class II molecules, it should be possible to detect the simultaneous binding of a stretch of protein to two MHCII alleles that have non-overlapping epitopes on the same protein by BIAcore surface plasmon resonance instrument. Preformed Biotinylated DR4 in complex with denatured H5N1-rHA1 was immobilized on streptavidin-coated (SA) BIAcore chip, followed by the injection of receptive DR1 in the presence of DM ( Fig. 6c ). The binding of DR1 to the complexes of DR4/H5N1-rHA1 produced 778 Response Unit RU signal. Injection of compact folded HA(306–318) bound DR1 (as negative control) produced 199 RU. This level of binding of DR1/HA(306–318) sample to HA1 protein is due to the presence of some empty DR1 molecules that were not in complex with HA(306–318) and were helped by DM. Binding of peptide-receptive DR1 to the complexes of DR4/H5N1-rHA1 indicates that more than one MHC class II molecules are capable of binding to the H5N1-rHA1 protein. Thus; (a) MHC class II molecule can bind to protein antigens, (b) just like peptide binding, DM enhances binding of full-length protein to DR1 and (c) binding of protein to DR1 occurs through peptide-binding groove of DR1 rather than other possible sites. Autoantigens are less susceptible to cathepsins So far, we have observed that immunodominant epitopes are either DM sensitive but cathepsin insensitive, or DM resistant but cathepsin sensitive. To expand our sample size, we examined few more autoantigens known to induce autoimmune diseases; uveitis-associated epitopes from retinal antigens, autoimmune thyroiditis-associated epitope from thyroglobulin and myocarditis inducing myosin heavy chain-α. Retinal arrestin (soluble-Ag (S-Ag)) is the antigen that is thought to be involved in uveitis in human and also in murine experimental autoimmune uveitis (EAU). Immunodominant epitope of retinal arrestin has been identified as hSA(291–306) (ref. 29 ), which induces EAU in HLA-DR3 (HLA-DRB1*03:01) transgenic mice. Thyroglobulin peptide, Tg(2,098–2,112), has been identified as an immunodominant epitope that induces murine experimental autoimmune thyroiditis in DR3-bearing transgenic mice [30] . Myosin heavy chain-α epitope, Myosin(334–352), has been shown to induce myocarditis in A/J mice [31] . To test cathepsin sensitivity, synthetic hSA(291–306), Tg(2,098–2,112) and Myosin(334–352) peptides were directly exposed to the cathepsin mixture and the reaction products were analysed. We found that hSA(291–306) and Tg(2,098–2,112) lacked the susceptibility to cathepsin digestion while being resistant to DM-mediated dissociation. 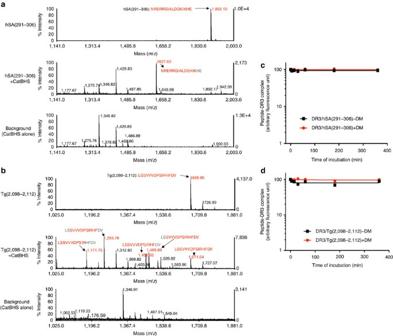Figure 7: HLA-DR3 binding core region of autoantigen-derived immunodominant epitopes shows resistance to the cathepsins and HLA-DM. (a,b) Mass spectra of retinal arrestin derived dominant epitope, hSA(291–306) and thyroglobulin-derived dominant epitope, Tg(2098–2112), after digestion with the cathepsins. Untreated synthetic peptides (a) hSA(291–306) or (b) Tg(2098–2112) are shown on the top spectra inaandb. Peptides were incubated with cathepsin B, H and S for 1 h at 37 °C (shown in the middle spectra). Background controls that included cathepsins alone are shown in the bottom spectra. The experiments were repeated twice. (c,d) Dissociation kinetics of fluorescently labelled hSA(291–306) or Tg(2,098–2,112) from DR3. (c) FL-hSA(291–306)/DR3 or (d) FL-Tg(2098–2112)/DR3 complexes were formed over a 3-day incubation with peptides in 37 °C and the unbound peptides were removed by spin column separation. Dissociation experiments were in the presence of 100 μM unlabelled hSA(291–306) or 100 μM unlabelled Tg(2,098–2,112) peptides at 37 °C for the indicated time in the presence (circle) or absence (square) of DM. The fluorescence of the labelled complex before dissociation was arbitrarily assigned a value of 100.0, and fluorescence after dissociation is expressed as a fraction of fluorescence before dissociation. Dissociation experiments were repeated twice. Figure 7a, top panel shows undigested hSA(291–306) at m/z 1,892 Da. On digestion with cathepsins, the full-length peptide peak at m/z 1,892 Da was minimized and a new peptide peak was detected at m/z 1,627 Da ( Fig. 7a , middle) and sequenced as NRERRGIALDGKIK that is missing two amino acids off of the C terminus. Other peptides detected at m/z 1,177, 1,275, 1,346, 1,429 and 1,487 Da were also detected in the background sample. Importantly, the loss of the two C-terminal residues does not abrogate the ability of this peptide to induce EAU in mice [29] . Figure 7: HLA-DR3 binding core region of autoantigen-derived immunodominant epitopes shows resistance to the cathepsins and HLA-DM. ( a , b ) Mass spectra of retinal arrestin derived dominant epitope, hSA(291–306) and thyroglobulin-derived dominant epitope, Tg(2098–2112), after digestion with the cathepsins. Untreated synthetic peptides ( a ) hSA(291–306) or ( b ) Tg(2098–2112) are shown on the top spectra in a and b . Peptides were incubated with cathepsin B, H and S for 1 h at 37 °C (shown in the middle spectra). Background controls that included cathepsins alone are shown in the bottom spectra. The experiments were repeated twice. ( c , d ) Dissociation kinetics of fluorescently labelled hSA(291–306) or Tg(2,098–2,112) from DR3. ( c ) FL-hSA(291–306)/DR3 or ( d ) FL-Tg(2098–2112)/DR3 complexes were formed over a 3-day incubation with peptides in 37 °C and the unbound peptides were removed by spin column separation. Dissociation experiments were in the presence of 100 μM unlabelled hSA(291–306) or 100 μM unlabelled Tg(2,098–2,112) peptides at 37 °C for the indicated time in the presence (circle) or absence (square) of DM. The fluorescence of the labelled complex before dissociation was arbitrarily assigned a value of 100.0, and fluorescence after dissociation is expressed as a fraction of fluorescence before dissociation. Dissociation experiments were repeated twice. Full size image We next examined thyroglobulin (2,098–2,112) peptide for its cathepsin sensitivity, which is detected at m/z 1,669 Da ( Fig. 7b , top). Cathepsin-exposed peptide produced truncated versions of the epitope at m/z 1,171 Da (LSSVVVDPSIR), 1,255 Da (SVVVDPSIRHF), 1,456 Da (LSSVVVDPSIRHF) and 1,469 Da (SVVVDPSIRHFDV), along with the reduced intensity of intact peptide at m/z 1,670 Da ( Fig. 7b , middle). To test the sensitivity of hSA(291–306) and Tg(2,098–2,112) to DM-mediated dissociation, we measured the dissociation kinetics of fluorescein-hSA(291–306) and fluorescein-Tg(2,098–2,112) in complex with DR3 in the presence or the absence of DM. DM functionality was tested in a binding assays ( Supplementary Fig. 4 ). When tested for DM sensitivity, DM did not facilitate the dissociation of either hSA(291–306) or Tg(2,098–2,112) from DR3 ( Fig. 7c,d ). These results suggest that these autoantigen-derived epitopes are selected as immunodominant by having two advantages—resistance to cathepsin digestions and resistance to DM-mediated dissociation. Sensitivity of Myosin(334–352) to cathepsin digestion was examined as with hSA and thyroglobulin peptides. While the majority of Myosin(334–352) remained intact after cathepsin digestion, minor fractions of shortened epitopes were also detected ( Supplementary Fig. 5 ). Next, we examined Myelin basic protein, MBP(84–102) that has been considered as a potential immunodominant epitope in relation to multiple sclerosis restricted to HLA-DR2b (DRB1*15:01) (ref. 32 ) and insulin B7-23 epitope, a candidate antigen for the induction of diabetes in NOD mice [33] . When MBP(89–101) peptide was directly exposed to the cathepsin mixture, although some trimming occurred, the major epitope, VHF F KNIVTPR at m/z 1,357 Da maintained its corresponding anchor residues for binding to DR2b. Interestingly, two shorter peptide fragments, F F KNIVTPR at m/z 1,121 Da and HF F KNIVTPR at m/z 1,258 Da, maintained at least some of their anchors including the major P4 fitting residues ( Supplementary Fig. 6 ) [34] , [35] . MBP(89–101) peptide has been reported to have two registers for binding to DR2a and DR2b. One of the shorter peptides shown lost P1 anchor for binding to DR2b, and the other lost P9 anchor for binding to DR2a. MBP(89–101) epitope is sensitive to DM-mediated dissociation [36] , hence the lack of sensitivity to cathepsins allows immunodominance. Similar to MBP peptide, digestion of insulin peptide at m/z 1,774 Da by the cathepsin mixture did not destroy the peptide ( Supplementary Fig. 7 ). The only other fragment detected post digestion of insulin B7-23 was a previously described epitope register for binding to I-A g7 (refs 37 , 38 , 39 ). In all, the trend seems to hold that immunodominant autoantigens are less susceptible to cathepsin digestion as compared with dominant epitopes from external pathogens ( Table 1 ). Table 1 Optimization of the reaction conditions for 4aa*. Full size table A destructive potential of CatD in MHCII antigen processing has been reported [40] . In light of resistance to our cathepsin mix, it was of interest to evaluate whether CatD or CatE might destroy the dominant epitopes from autoantigens during antigen processing and epitope selection. We tested this potential in a cellular IFN-γ ELISPOT assay in combination with pharmacological inhibitors of CatD/E, Pepstatin A and a cell-penetrating variant of it, Pepstatin A-Penetratin (PepA-P) [41] . The results depicted in Supplementary Fig. 8 indicate that the inclusion of PepA or PepA-P did not significantly reduce the generation of immunodominant epitopes of three antigens tested; recombinant influenza HA1, influenza H5N1 and collagen II. This was in sharp contrast to the complete inhibition of the dominant epitope generation in the presence of CatB inhihitor, CA-074ME, in agreement with data mentioned above. We conclude that CatD/E may not have a critical role in generation of immunodominant epitopes during MHC class II antigen processing, although further experiments would be necessary to exclude this possibility. DM increases the abundance of dominant epitope To find out how DM influences peptide selection, we compared two parallel samples assembled for processing of H5N1-rHA1 with or without DM. The immunodominant peptide at m/z 1,814 Da was detected in both samples and that the repertoire of eluted peptides remained unchanged, although, the intensity of m/z 1,814 Da peak was higher in the presence of DM ( Fig. 8 ). To evaluate the relative quantities of the peak in two samples, we used selected reaction monitoring. Label-free mass spectrometry methods for relative quantitation of MS peaks have the advantage of experimental simplicity and applicability. In label-free quantitation, protein profiling comparisons are based on the relative intensities of extracted ion chromatograms. This approach therefore does not require any metabolic, chemical and enzymatic labelling [42] , [43] . 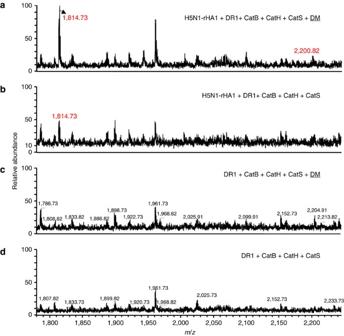Figure 8: Repertoire of H5N1-rHA1-derived peptides appears the same with or without DM. Samples containing equal starting materials (same amount of DR1 and rHA1 protein) were prepared in the presence, or absence of DM and the eluted peptides were analysed by MALDI. (a–d) Native form of H5N1-rHA1 protein, DR1, and the cathepsins B, H and S were incubated in the (a) presence or (b) absence of DM. (c) and (d) are background spectra for samplesaandb, respectively, from reactions not containing H5N1-rHA1. Immunodominant epitopes, HA(259–274) (SNGNFIAPEYAYKIVK), and HA(259–278) (SNGNFIAPEYAYKIVKKGDS), are shown atm/z1,814.7 and 2,200.8 Da. The experiments were repeated three times. Figure 8: Repertoire of H5N1-rHA1-derived peptides appears the same with or without DM. Samples containing equal starting materials (same amount of DR1 and rHA1 protein) were prepared in the presence, or absence of DM and the eluted peptides were analysed by MALDI. ( a – d ) Native form of H5N1-rHA1 protein, DR1, and the cathepsins B, H and S were incubated in the ( a ) presence or ( b ) absence of DM. ( c ) and ( d ) are background spectra for samples a and b , respectively, from reactions not containing H5N1-rHA1. Immunodominant epitopes, HA(259–274) (SNGNFIAPEYAYKIVK), and HA(259–278) (SNGNFIAPEYAYKIVKKGDS), are shown at m/z 1,814.7 and 2,200.8 Da. The experiments were repeated three times. Full size image Fresh samples containing equal starting materials (same amount of DR1 and rHA1 protein) were prepared in the presence or absence of DM and the eluted peptides were analysed by liquid chromatography tandem mass spectrometry. The m/z 1,814 Da peak of HA(259–274) was detected by matrix-assisted laser desorption/ionization (MALDI) first ( Fig. 8 ). For relative quantification of this peptide, the samples were run on LTQ mass spectrometry and HA(259–274) was detected as doubly charged ions at m/z 907 Da. The MS2 profile of the doubly charged ions produced two major daughter ions at m/z 1,110 and 1,181 Da ( Fig. 9a ). The peak area values from extraction ion chromatograms of 1,110 or 1,181 Da daughter ions in samples with or without DM are shown in Fig. 9b,c and were estimated as 3,356 and 3,064 in the presence of DM, versus 626 and 597 without DM accordingly. Both daughter ions showed greater area and higher intensities in the presence of DM. None of those daughter ions were detected in the background samples. Thus, H5N1-rHA1-derived HA(259–274) was enriched in the presence of DM by about five-folds. These data suggests that DM influences the amount of epitopes captured by DR1. 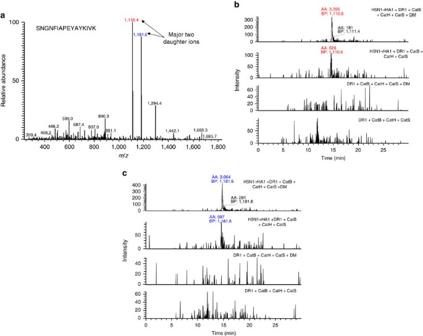Figure 9: DM increases the abundance of dominant epitope. Quantitation of HA(259–274) epitopes obtained in samples with or without DM by liquid chromatography (LC) combined with Linear Ion Trap Quadrouple tandem mass spectrometry (LC-LTQ MS/MS). Samples containing equal starting materials (same amount of DR1 and rHA1 protein) were prepared in the presence or absence of DM and the eluted peptides were analysed. For relative quantification of this peptide, the samples were rerun on LTQ mass spectrometry and HA(259–274) was detected as doubly charged ions atm/z907 Da. (a) The MS/MS profile of the doubly charged ions produced two major daughter ions atm/z1,110 and 1,181 Da. (b) The base peak area values from extraction ion chromatograms of 1,110 or (c) 1,181 Da daughter ions in samples with or without DM are shown and were estimated as 3,356 and 3,064 in the presence of DM, versus 626 and 597 without DM accordingly. Neither of those daughter ions were detected in the background samples. (AA, automated area calculated using Genesis peak detection algorithm; BP, base peak). The experiments were repeated twice and each experiment was quantified two times. Figure 9: DM increases the abundance of dominant epitope. Quantitation of HA(259–274) epitopes obtained in samples with or without DM by liquid chromatography (LC) combined with Linear Ion Trap Quadrouple tandem mass spectrometry (LC-LTQ MS/MS). Samples containing equal starting materials (same amount of DR1 and rHA1 protein) were prepared in the presence or absence of DM and the eluted peptides were analysed. For relative quantification of this peptide, the samples were rerun on LTQ mass spectrometry and HA(259–274) was detected as doubly charged ions at m/z 907 Da. ( a ) The MS/MS profile of the doubly charged ions produced two major daughter ions at m/z 1,110 and 1,181 Da. ( b ) The base peak area values from extraction ion chromatograms of 1,110 or ( c ) 1,181 Da daughter ions in samples with or without DM are shown and were estimated as 3,356 and 3,064 in the presence of DM, versus 626 and 597 without DM accordingly. Neither of those daughter ions were detected in the background samples. (AA, automated area calculated using Genesis peak detection algorithm; BP, base peak). The experiments were repeated twice and each experiment was quantified two times. Full size image Our reductionist system for MHC class II molecules composed of only five soluble purified components has proved to be sufficient for antigen processing and the selection of immunodominant epitopes. Because of its defined nature, this system can lend itself to elucidating steps involved in antigen processing and deciphering molecular mechanisms involved in epitope selection. Here we examined four antigens from pathogens and six autoantigens, known for their role in autoimmune diseases, and found clear differences in processing of the two types of antigens. We show that prior digestion of external proteins with cathepsins eliminates the capture of immunodominant epitope by HLA-DR; conversely, if the antigen is first captured by HLA-DR in the presence of HLA-DM, dominant epitopes are selected successfully. A different picture emerged for examples of autoantigens. We learned that epitopes from autoantigens were less sensitive to destruction by the enzymes in the system. In fact, the core sequences of the dominant epitopes of autoantigens were mostly resistant to cathepsin digestion. Two major hypotheses regarding antigen-processing pathways have been put forward by Trombeta and Mellman [44] . In one model, ‘bind first, cut/trim later’, described by Sercarz proposes that MHC molecules scan the length of protein antigens to find the best fitting epitopes [2] . On the basis of the second model, peptides are cut first and then chosen for presentation to T cells. Our findings here comply with both models. With respect to the antigens from external sources, our data fits the former model, but with respect to autoantigens the latter model is more suitable. A number of studies support bind first, cut later model: a single cut by AEP in tetanus toxoid facilitated presentation of the dominant epitope to specific T cells [45] . Mimura et al . [46] provided evidence for the ‘bind first, cut/trim later’ model for a tumour antigen, Sette et al . [47] showed denatured proteins binds MHCII, Runnel et al . [48] demonstrated that protein binding to MHC was enhanced by DM and Castellino et al . [49] provided evidence for binding of both I-A k and I-E k molecules to HEL. Consistent with ‘binding first, trimming later’ model, accessibility of dominant epitopes for binding to MHCII is another parameter that might contribute to preferred epitope selection during antigen processing [50] . In our system, the HA(306–318) epitope is located at the C terminus of the rHA1 possibly offering an advantage for its capture by MHCII; it forms DM-resistant complexes with DR1. Accordingly, HA(306–318) will be protected from proteolysis and will be displayed at a higher abundance relative to other potential epitopes that are located further away from the protein termini. This might explain why many known immunodominant epitopes are located at the C or N termini [51] , [52] , [53] or on flexible strands of protein antigens [50] . A popular model for epitope selection is the intrinsic affinity of peptide for MHC II [7] , although there are also a number of publications that report lack of correlations between binding affinity and immunodominance [20] , [54] , [55] . It has now been documented that a peptide/DR1 complex that has an empty or partially filled P1 pocket is a favourable substrate for interaction with DM, whereas a compact and rigid conformation with filled P1 pocket is an unfavourable substrate [13] , [56] . The autoantigen-derived epitopes we tested resisted digestion by the cathepsins in the system. Because of reliance of autoimmune epitopes on cathepsins, it is possible to hypothesize that such epitopes would not be generated in the thymus and thus T cells reactive to them would not be deleted [37] . In the periphery, however, it is likely that autoantigens are generated in extracellular matrix where many proteases are already at work, and that only epitopes that survive such milieu may get a chance to be further processed and presented by APCs. A member of the family of matrix metalloproteinases is gelatinase B (MMP-9) that is known for its role in generating collagen II fragments supports this interpretation [57] . It is fair to say that under inflammatory conditions generated by infections or other causes, collagen fragments are generated by MMP-9 and are picked up by the APCs, which process and present them to the T cells. Despite being sensitive to DM-mediated dissociation, but because of its resistance to the cathepsins, collagen epitope can rebind to the MHCII and presented. Another example we tested was the thyroglobulin dominant epitope, which has been reported to induce thyroiditis. It is documented that this epitope is proteolysed in the thyroid tissue by multiple cathepsins at neutral pH and then is taken up by the APCs [30] , [58] . We showed that the DR3 binding core of this epitope is resistant to further cleavage by the cathepsins. A third example we tested was a uveitis (EAU)-inducing peptide, which was reduced by two residues at its C terminus, which did not reduce its effectiveness in inducing EAU in DR3 transgenic mice [29] . Both EAU and thyroglobulin dominant epitopes were resistant to DM-mediated dissociation, suggesting that autoantigens may or may not be DM sensitive. We also tested a DR2-restricted MBP(84–102) peptide, which followed the same trend as the other autoantigens tested. Interestingly, it has been reported that MBP is a substrate for CatS digestion, although the major cutting sites fall outside the core of immunodominant epitope of MBP. It is only under extreme conditions, that is, 20 h incubation with CatS, the immunodominant epitope might also be cut [59] . Clearly, there are many cathepsins in the cellular environment but not all are involved in the generation and selection of the dominant epitopes, and/or have redundant roles. In addition, activities of cathepsins are tightly regulated [5] , [60] , [61] and vary by cellular activity or maturation. CatD and E have been proposed to have destructive roles for myoglobin presentation [40] . We tested whether the inhibition of CatD/E in cells would affect the presentation of dominant epitopes in three of our antigens, and it appeared that the effect if any was incremental. While CatD/E do not appear to have a major role in dominant epitope selection for the antigens tested here, it is possible that they may be involved in the processing of other antigens. Only further experiments can attest their contributions to epitope selection. Our model was verified by testing vaccinia epitope I6L(338–352) that has previously been identified as an immunogenic epitope using peptide elution studies from DR1-expressing DC [62] . Exposure to our standard cathepsins destroyed this peptide leaving a cleavage product, SSFPVPT, which was too short to bind DR1 stably. Moreover, when examined for DM-mediated sensitivity, I6L(338–352)/DR1 complex was DM sensitive ( Supplementary Fig. 9 ). According to our model, I6L(338–352) cannot be an immunodominant epitope as it is sensitive to both cathepsins and DM. Indeed, this epitope did not generate a primary response in CD4 T cells from DR1 + individuals; only after a boost, T cells responded to this peptide moderately [62] . Using our cell-free antigen-processing system, we have presented data to indicate that there are at least two different paths for processing of dominant epitopes that are derived from autoantigens versus pathogen-derived antigens. We find that both cathepsin sensitivity and DM sensitivity play key roles in determination of immunodominance. Contribution of endosomal proteases, CatB, CatH and CatS, combined with DM effects critically influence the repertoire of peptides captured by DR molecules. Indeed, we have obtained evidence for the significance of CatB and CatS in the processing of H5N1-rHA1 and collagen II proteins for presentation of H5N1-HA(259–274) and CII(280–294) epitopes ex vivo . Using a specific chemical inhibitor of CatB [19] , we find that processing and presentation of HA(259–274) and CII(280–294) epitopes were completely inhibited in cytokine production by specific T cells in culture. The two paths can be described as (a) immunodominant epitopes are selected by DM and retained by DR molecules, while epitopes that are DM sensitive are removed and destroyed by the cathepsin or (b) for autoantigens tested here, cathepsin resistance is the key determinant while DM sensitivity can be an added advantage, but is not an absolute necessity. Importantly, the non-dominant epitopes are sensitive to both DM and cathepsins: DM dislodges those epitopes from the MHCII groove, and the cathepsins destroy them. The net result is that most of the MHC molecules will end up with epitopes that are bound to MHCII very tightly, or not so tightly, but because of resistance to digestion by the cathepsins they are dislodged by DM and can rebind. The important net result of all these events is that the immunodominant epitopes gain relative abundance, as we have shown by quantitative MS and as suggested for cellular processing [54] . Production of recombinant proteins Soluble DR1*01:01 was produced as described [12] . In brief, bacculovirus DNA (BaculoGold; PharMingen) and transfer vectors carrying DR α- and β-chain genes were transfected together into Sf9 insect cells to produce recombinant viruses. Hy5 cells were infected with the recombinant viruses and DR1 proteins were purified from culture supernatants with immunoaffinity chromatography columns with monoclonal antibody L243 to DR1 (purified from HB-55 hybridoma; American Type Culture Collection). Soluble HLA-DM was expressed by Hy5 cells transduced with recombinant bacculovirus containing extracellular domains of the genes encoding the α- and β-chains of human HLA-DM. The truncated DM α- and β-chains were genetically modified to contain the Flag epitope (DYKDDDDK) and the c-Myc epitope (EQKLISEEDL), respectively, at their C termini. Protein was purified from culture supernatants with monoclonal antibody to M2 (anti-Flag) sepharose resin (Sigma), was eluted with 0.1 mg ml −1 of Flag peptide in 0.05% (w/v) sodium azide in PBS, was further purified by gel-filtration chromatography (Superdex 200 HR 10/30 column; Amersham Pharmacia) and was stored at –80 °C at a concentration of about 1 mg ml −1 in 0.05% (w/v) sodium azide in PBS. rHA1 was produced as described previously in E. coli [18] . H5N1-rHA1 from strain A/Vietnam/1203/2005, purified from 293 cells, was purchased from commercial sources (eEnzyme, Gaithersburg, MD, USA). H5N1-HA protein was obtained from BEI Resources. Biotinylated HLA-DR4 (DR4)/CLIP and HLA-DR3 (DR3)/CLIP were obtained from NIH Tetramer Core Facility (Atlanta, GA). Bovine type II collagen (bCII) was purchased from Chondrex (Chondrex, Redmond, WA, USA). Peptides synthesis and peptide labelling Peptides human CLIP, hCLIP(89–105), KMRMATPLLMQALPM, HA(Y308A), PKAVKQNTLKLAT, CII(280–294), CAGFKGEQGPKGEPGP OH and CII(954–968) 2OH , FTGLQGLP OH GPP OH GPSGC were synthesized by Global Peptide (currently Pi Proteomics, Huntsville, AL, USA). HA(306–318) peptide, PKYVKQNTLKLAT, H5N1-HA(259–274), SNGNFIAPEYAYKIVK, MBP(89–101), CVHFFKNIVTPRTP and hSA(291–306), NRERRGIALDGKIKHE, were synthesized by Elim Biopharmaceuticals Inc. Thyroglobulin peptide Tg(2,098–2,112), LSSVVVDPSIRHFDV, was synthesized by GenScript Inc. All peptides were at 90–95% purity as analysed by reverse-phase high-performance liquid chromatography, and their identities were confirmed by mass spectrometry. Tg(2,098–2,112) and hSA(291–306) were fluorescently labelled at N termini [27] . Fluorescent labelling of CII peptides was through an added N-terminal cysteine as described previously [12] . Peptide binding and dissociating assays Before setting up the peptide-binding assays [62] , DR3/CLIP complexes were thrombin cleaved for 1 h at room temperature (Thrombin was purchased from Novagen, EMD Millipore chemicals, Billerica, MA, USA). After the thrombin cleavage, 500 μM phenylmethylsulfonyl fluoride (Sigma-Aldrich, St Louis, MO, USA) was added to inactivate the enzyme. For binding assays, DR3 (1 μM) was incubated for various times in the presence or absence of 1 μM DM together with 50 μM fluorescence-labelled peptides in citrate-phosphate buffer (pH 5.0) at 37 °C. Unbound peptide was removed by spin columns (Sephadex G-50 equilibrated with PBS/0.1% filtered non-fat milk) at pH 7.4. Fuorescence emission of the fluorescein isothiocyanate–peptide–DR complexes was measured at 25 °C and 514–516 nm with excitation at 492 nm on a Fluoromax3 spectrofluorometer (Horiba Jobin-Yvon, Kyoto, Japan) with a slit width of 2 nm. For dissociation assays, a stock solution of DR1 or DR3 (10 μM) was incubated with fluorescence-labelled peptide (150 μM) in PBS/NaN 3 for 3 days at 37 °C to yield maximal loading. Unbound fluorescent peptide was removed by spin columns. Dissociation of fluorescent peptide/DR complexes (1 μM) was monitored in samples incubated for different length of times in the presence of excess unlabelled competitor peptide (100 μM) with or without DM. Fluorescence signal was measured after one more spin column separation as described above. Proliferation and cytokine assays HLA-DR1 (DRB1*0101) transgenic mice (originally obtained from Dr Denis Zaller, Merck) expressing a fusion product of the DR1 binding groove and the membrane proximal domain of I–E molecules [21] were backcrossed to MHC class II KO mice for 12–16 generations to eliminate endogenous class II proteins (I-A f ) and then were inbred to homozygocity. DR1-transgenic mice were immunized with 100 μg type II collage proteins or peptides in CFA at the base of the tail. After 8–10 days, cells were harvested from the draining lymph nodes and incubated with a range of peptide and protein concentrations for 3 days in culture before adding [ 3 H] thymidine (Amersham). Cells were then harvested and counted after a further 18–20 h culture. For cytokine assays, the draining lymph nodes of the immunized mice were collected after 10 days and cells (5 × 10 5 ) were incubated with a range of peptide and protein concentrations. Culture supernatants were collected 48 h later and IL-2 concentrations were measured by enzyme-linked immunosorbent assay (ELISA) (R&D System). The optical density was measured in an ELISA reader (Dynex Technologies) at 450 nm and a reference wavelength of 570 nm. For IFN-γ ELISPOT assay (BD Biosciences), cells (8 × 10 5 ) from the draining lymph node were incubated with peptides (5 μM), or proteins (0.25 μM) for 24 or 48 h in the presence or absence of cathepsin inhibitor, CA-074ME (Calbiochem), (5–10 μM), Pepstatin A (Sigma) (100–200 μM) or Pepstatin A-Penetratin (Calbiochem), (10–20 μM),. After the incubation, ELISPOT plate was analysed with the CTL Immunospot Analyzer plate reader and software (Cellular Technology Limited). Gentle SDS–PAGE assay Samples were prepared by incubating DR1 (1 μM) with various combinations of the following: rHA1 (2.7 μM), HA(306–318) (300 μM) and DM (1 μM) in citrate-phosphate buffer pH 5.0/0.05% NaN 3 for 3 h in 37 °C waterbath. Following incubation, pH was adjusted to 7.4 with either 0.2 M sodium phosphate dibasic or 1 M Tris-HCl pH 8.0 and the samples were mixed with a modified Laemmli buffer with 0.1% SDS final concentration and no reducing agents. The samples were resolved without boiling on 12% polyacrylamide gels and were silver stained [63] . For western blot experiments, various combinations of DR1(1 μM), DM (0.5 μM), rHA1 (2 μM) or HA(306–318) (300 μM) were incubated in citrate-phosphate buffer pH 5.0 overnight at 37 °C. The pH was readjusted to 7.4 and the samples were mixed with Laemmli buffer containing 0.1% SDS and 2.5% 2ME. They were either not boiled (room temperature) or boiled before loading on 10% SDS–PAGE. Samples on gel were transferred to PVDF membranes; DR1/protein complexes were detected by anti-His mAb (1:10,000) (Invitrogen) or CHAMP2 (1:4,000) (Rabbit polyclonal anti-DR1 serum (Gift from Dr Larry Stern), followed by staining with anti-mouse HRP (1:5,000) or anti-Rabbit HRP Ab (1:5,000) respectively. Surface plasmon resonance experiments Biotinylated DR4/CLIP was thrombin cleaved for 1 h at room temperature and incubated with 100-folds molar excess of HA(Y308A) for 3 days at 30 °C to generate peptide-receptive DR4. After removing unbound HA(Y308A) by spin column filtration equilibrated in PBS/0.05% NaN 3 , DR4-HA(Y308A) (5 μM) complexes were incubated with denatured H5N1-rHA1 protein (eEnzyme) (2 μM) and DM (1 μM) for 20 min at 37 °C. Immediately after, DR4-H5N1-rHA1 protein complexes were injected over Sensor chip SA (streptavidin) (GE Healthcare Biosciences, Waukesha, WI, USA). Receptive DR1 (incubated with excess HA(Y308A) for 3 days at 37 °C) or HA(306–318) bound DR1 (2 μM) (closed DR1) were injected over H5N1-rHA1 bound DR4 immobilized surface in the presence of DM (1 μM). All protein solutions were diluted in the running buffer composed of citrate-phosphate pH 5.5 with 150 mM NaCl, 0.005% Tween-20 and 0.05% NaN 3 . Measurements were done at 37 °C with flow rates ranging between 1–3 μl min −1 . Binding sensograms were collected on a BIAcore 1,000 instrument (GE Healthcare Biosciences, Waukesha, WI, USA). Mass spectrometry Sample preparations for MS analyses . HLA-DR1, protein antigen and HLA-DM were incubated in citrate-phosphate buffer (pH 5.0–5.2) at 37 °C for 3 h before adding cathepsin B (bovine spleen, Sigma), cathepsin H (human liver, Calbiochem) and cathepsin S (human recombinant produced in E.coli , Calbiochem) in 6 mM L -Cysteine and 4 mM EDTA for an additional 2–3 h. For synthetic peptide digestion samples, peptides were incubated in citrate-phosphate buffer (pH 5.0) at 37 °C for 1 h with cathepsins B, H and S and 6 mM L -cysteine and 4 mM EDTA. For some experiments with type II collagen and rHA1 proteins, only cathpesin B and H were added, while most experiments were done with all three cathepsins, B, H and S. After digestion, the pH was adjusted to 7.4, 10 μM iodoacetamide was added and DR1 was immunoprecipitated with HLA-DR-specific mAb (L243)-conjugated Sepharose beads. Bound peptide was eluted with trifluoroacetic acid (TFA) (1%) and filtered through a 10-kDa MWCO Microcon (Millipore) and lyophilized. Samples from synthetic peptide digestions were filtered through a 10-kDa MWCO Microcon, washed with 10% MeOH/0.1% TFA and lyophilized. Lyophilized filtrates were resuspended in 10 μl 0.1% TFA and zip tipped (Millipore) for analysis by mass spec. vMALDI-LTQ XL analysis . Lyophilized samples were resuspended in 5–10 μl 50% ethanol/50% water/0.2% TFA. Resuspended (0.5 μl) sample was spotted, dried and covered with 0.5 μl matrix (either 2,5-Dihydroxybenzoic acid, 40–50 mg ml −1 in 50% ethanol/50%water/0.15%TFA or α-Cyano-4-hydroxycinnamic acid, 2.5 mg ml −1 in 50% ethanol/50% water/0.15% TFA). First Full MS (1,100–4,000 Da mass range) was acquired on a vMALDI-LTQ XL (Thermo Fisher Scientific) and then MS2 and MS3 CID (collision-induced dissociation) spectra were acquired on peptides of interest. Spectra were manually acquired using CPS plate motion, 2 microscans, 0 sweep scans, automatic gain control (AGC) feature ‘on’, automatic scan filtering ‘on’ and set on 3,000 for Full MS and 200 for MSn, and accumulating 10–15 scans for Full MS and 15–25 scans for MSn. Data analysis . Full MS spectra were first visually scanned to find peptides of interest. MSn data collected for the peptides of interest were searched with Bioworks 3.3.1 SP1 (Thermo Fisher) against a custom-built database. The custom database contained protein sequences of all components presented in the sample reactions. MSn data was searched with the following parameters; no enzymes, monoisotopic precursor and fragment ions, two missed cleavage sites, peptide tolerance of 1-2 Da, fragment ion tolerance of 1 Da and variable modifications including carboamidomethylated cysteine, oxidized methionine and methionine with 48 Da loss for MS3. LTQ analysis for relative quantification of H5N1-rHA1 immunodominant epitope . Lyophilized samples were resuspended in water/1% TFA/0.2% acetonitrile; 5 μl was loaded on nano-LC-ESI/MS/MS platform connected to LTQ XL (ThermoFisher) interfaced with a 2D nanoLC system (Eksigent, www.eksigent.com ). Peptides were fractionated by reverse-phase high-performance liquid chromatography on a 75 μm × 100 mm C18 column (YMC ODS-AQ 5 um particle size, 120 Å pore size) with a 10 μm emitter (New Objective) using 10–40% acetonitrile/0.1% formic acid gradient at 300 nl min −1 over 15 min time. Using selected reaction monitoring two transitions, 907.6 Da to 1110.5 (±1.0 Da) and 907.6 to 1181.5 (±1.0 Da) were monitored using 2.2 kV source voltage, collision energy of 35 V, Q =0.250; activation time=30. How to cite this article: Kim, A. et al . Divergent paths for the selection of immunodominant epitopes from distinct antigenic sources. Nat. Commun. 5:5369 doi: 10.1038/ncomms6369 (2014).